Self-assembly of two-dimensional DNA origami lattices using cation-controlled surface diffusion DNA origami has proven useful for organizing diverse nanoscale components into patterns with 6 nm resolution. However for many applications, such as nanoelectronics, large-scale organization of origami into periodic lattices is desired. Here, we report the self-assembly of DNA origami rectangles into two-dimensional lattices based on stepwise control of surface diffusion, implemented by changing the concentrations of cations on the surface. Previous studies of DNA–mica binding identified the fractional surface density of divalent cations as the parameter which best explains the behaviour of linear DNA on mica. We show that for between 0.04 and 0.1, over 90% of DNA rectangles were incorporated into lattices and that, compared with other functions of cation concentration, best captures the behaviour of DNA rectangles. This work shows how a physical understanding of DNA–mica binding can be used to guide studies of the higher-order assembly of DNA nanostructures, towards creating large-scale arrays of nanodevices for technology. DNA allows the programmed self-assembly of two- [1] , [2] and three- [3] , [4] , [5] , [6] dimensional (2D and 3D) nanoscale shapes and patterns, whose resolution cannot yet be matched by top-down fabrication. DNA origami, in particular, has proven useful for organizing nanoscale objects, such as biomolecules [7] , [8] , [9] , nanoelectronic or photonic components [10] , [11] , [12] , small molecules [13] and moving DNA machines [14] , [15] , [16] . While an individual origami can serve as a template for up to 200 small devices, typically only a single multi-component electronic or optical device is constructed [10] , [12] . For many technological applications it would be desirable to organize origami into periodic arrays, for example, to allow wiring of electronic devices together, to create cooperative optical effects as seen in optical metasurfaces [17] , to create DNA ‘etch masks’ [18] , [19] or to enable easier extraction of single-molecule biophysical data [9] , [20] . Directed self-assembly of individual DNA origami using arrays of lithographically patterned sticky patches is one approach [21] , [22] , [23] ; however, it requires numerous fabrication steps, very high resolution e-beam or nanoimprint lithography and careful control of deposition. Solution synthesis of periodic DNA origami lattices is being explored [24] , [25] , and transfer of solution-assembled lattices onto substrates is another potential approach. However, the reliable deposition of large self-assembled DNA lattices from solution onto surfaces is challenging: lattices often break or distort as they are deposited. Assembling DNA lattices directly on substrates may provide a route to more reproducible patterning. Several studies have demonstrated that the annealing of small DNA tiles over mica or silicon dioxide can form large lattices [26] , [27] , [28] , but these lattices are comprised of ~10 nm tiles, which cannot be used to template complex multi-component devices. Such protocols are incompatible with origami because, under the divalent-cation-rich conditions used, origami (which are much larger than the tiles) are immobile and cannot diffuse to form lattices. Divalent cations, particularly Mg 2+ and Ni 2+ , have long been used to bind natural double-stranded DNA (dsDNA) [29] and artificial DNA structures to mica [30] and other substrates [21] . For artificial DNA nanostructures, cation-dependent mica binding has not been studied quantitatively. In particular, the competition between monovalent and divalent cations measured in biophysical studies [31] , [32] has not been considered, perhaps because it has been assumed that divalent cations dominate the DNA–mica interaction. Here we report the self-assembly of DNA origami into 2D checkerboard lattices based on a novel mechanism: stepwise control of surface diffusion mediated by exploiting the competition between Mg 2+ and Na + in DNA–mica binding. Understanding gained in optimizing lattice formation has allowed us to connect the self-assembly of artificial DNA nanostructures to biophysical observations of dsDNA surface diffusion, and we suggest that previously explored biophysical parameters are generally applicable to the interaction of artificial DNA nanostructures and mica. In particular, our exploration of several cation-dependent parameters indicates that in a high ionic strength ( I >0.4 M)/short Debye length regime ( λ D ≲ 0.45 nm), the fractional surface density of divalent cations, , best captures the conditions suitable for lattice formation. Notably, the bulk concentration of Mg 2+ is found to be the worst predictor of lattice formation. The onset of lattice formation behaves similar to a previously observed -determined strong-to-weak binding transition for circular dsDNA [32] , and may indicate an analogous transition for DNA origami on mica, one which enables surface diffusion. However the high strength of origami binding yields a transition at a lower value (~0.2 rather than ~0.65), and good lattice formation appears to require more than just surface diffusion since decreases lattice incorporation rates. We suggest how this and other effects may be explained by origami geometry. Finally, we describe the effect of mica inhomogeneities on the morphology of lattices, which suggests how better-defined lithographic substates might be used to control lattice size and orientation. Rectangle design and surface diffusion protocol To programme rectangular origami to form the desired checkerboard lattices, we designed them to form bonds via their four corners ( Fig. 1 ). Rather than using single-stranded sticky ends, bonds were mediated by blunt-end stacking interactions [33] . We chose stacking interactions for two reasons: first, to allow potential rearrangements during the surface assembly process via a putative sliding mechanism (sticky ends would have required unwinding and rewinding of the strands), and second, to achieve symmetry between the corners (with stacking bonds, two origami contacting via their corners would be able to bind regardless of their relative rotations). Both motivations reflected our desire to encourage the fast assembly of large lattices without kinetic trapping, although we did not test the importance of these design criteria in this work. 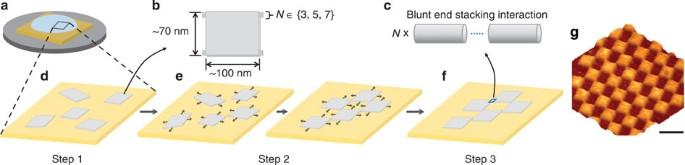Figure 1: Schematics for checkerboard-forming DNA rectangle design and surface diffusion protocol. (a) Assembly takes place on a mica surface (yellow) affixed to a steel disk (grey) under a drop of buffer (blue). (b) Rectangular origami (100 nm × 70 nm) have four potential binding interactions, one at each corner and each potential binding interaction is composed ofNblunt-end helices. (c) Each corner is capable of makingNblunt-end stacking interactions when origami bond. (d) Step 1, origami are deposited on mica at ionic conditions under which they are immobile (TAE/12.5 mM Mg2+). (e) Step 2, ionic conditions are changed to allow the origami to diffuse and form lattices over a 4-h incubation (~700 mM Na+is added, and the sample is optionally heated to 40 °C). (f) Step 3, ionic conditions are changed to stop diffusion and immobilize the resulting structures (first, ~1 mM Ni2+is added for a 5 min incubation; second, the buffer is exchanged to TAE/12.5 mM Mg2+to remove residual Na+). (g) A topographic AFM image of the resulting structure. Scale bar, 200 nm. Figure 1: Schematics for checkerboard-forming DNA rectangle design and surface diffusion protocol. ( a ) Assembly takes place on a mica surface (yellow) affixed to a steel disk (grey) under a drop of buffer (blue). ( b ) Rectangular origami (100 nm × 70 nm) have four potential binding interactions, one at each corner and each potential binding interaction is composed of N blunt-end helices. ( c ) Each corner is capable of making N blunt-end stacking interactions when origami bond. ( d ) Step 1, origami are deposited on mica at ionic conditions under which they are immobile (TAE/12.5 mM Mg 2+ ). ( e ) Step 2, ionic conditions are changed to allow the origami to diffuse and form lattices over a 4-h incubation (~700 mM Na + is added, and the sample is optionally heated to 40 °C). ( f ) Step 3, ionic conditions are changed to stop diffusion and immobilize the resulting structures (first, ~1 mM Ni 2+ is added for a 5 min incubation; second, the buffer is exchanged to TAE/12.5 mM Mg 2+ to remove residual Na + ). ( g ) A topographic AFM image of the resulting structure. Scale bar, 200 nm. Full size image Our surface diffusion protocol is based on biophysical studies, which demonstrated that changing the relative concentration of divalent and monovalent cations can profoundly change the surface mobility and reversibility of binding of long DNA on a mica surface [32] , [34] , [35] . To perform surface diffusion ( Fig. 1 ), we deposited origami on a mica surface under buffer conditions for which the origami are immobile (Step 1), changed the buffer condition to allow the origami to diffuse on the surface or within a confined layer near the surface (Step 2), and changed the buffer condition to again immobilize the origami for imaging (Step 3). For the initial deposition step, we used a buffer which was rich in the divalent cation Mg 2+ (1 × Tris-acetate-EDTA buffer (TAE) with 12.5 mM Mg 2+ ; this buffer is used for origami formation and atomic force microscopy (AFM), and it has a low monovalent concentration with [TrisH + ]≈15 mM. Calculation of the concentration of all ionic species for all buffers is explained in Supplementary Note 1 and summarized in Supplementary Table 1 ). Since monovalent cations are known to weaken the binding of DNA to mica [31] , [32] , [35] , [36] , we implemented the diffusion step by exchanging the buffer to one whose predominant cation is Na + (~700 mM NaCl). During the diffusion step, we also mildly heated samples at a constant temperature (40 °C, for ~4 h; while heating above room temperature appears to facilitate the process, it is not essential for the surface diffusion of origami; evidence provided later). Since Ni 2+ is known to bind DNA to mica more strongly than Mg 2+ does [29] , [37] , even in the presence of competing Na + ions [35] , we used it to implement the immobilization step. Adding concentrated Ni 2+ solution (yielding ~1 mM Ni 2+ in the sample) stopped diffusion and ‘froze’ the product structures onto the surface. After 5 min, the buffer was exchanged back to TAE/Mg 2+ for AFM imaging. We note that in general we do not expect the 4 h diffusion step to achieve thermodynamic equilibrium, particularly later when we examine ionic conditions having low origami mobility. However, we have observed that, under ionic conditions which achieve the best lattice formation, the distribution of lattices does not change much after 30 min. 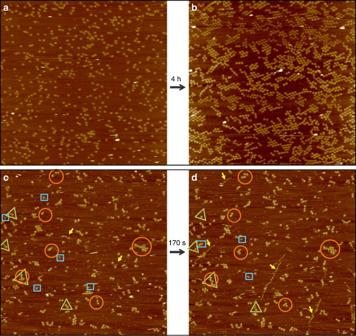Figure 2: DNA origami checkerboard lattices self-assembled by surface diffusion. (a,b) Before assembly (a) no lattices are observed by AFM, but after the surface diffusion protocol (b) 98.6% of rectangles (n=2,380) have been incorporated into lattices. Images inaandbare not from the same position on the mica surface, but are representative before/after images. (c,d) Consecutive AFM images show attachment events of origami to lattices (orange circles), detachment events (green triangles), movements of individual origami or small lattices which appear or disappear between frames (blue rectangles) and structures dragged by the AFM tip (yellow arrows). All images are 10 μm × 10 μm. Two-dimensional lattices assemble by surface diffusion Figure 2 shows the self-assembly of rectangular origami into checkerboard lattices by surface diffusion, as visualized by AFM. We first examined the assembly of origami with three blunt-end helices per potential bond ( N =3). After initial deposition of such origami on mica, we observed no lattices ( Fig. 2a ) and at most a few linear dimers per 100 μm 2 area. After our protocol ( Fig. 2b ), we measured the post-diffusion state of 2,380 origami rectangles and found that 98.6% of all rectangles were incorporated into lattices with an average size of 7.3±6.9 (s.d.) origami per lattice. We suggest that electrostatic confinement of origami to the surface thermodynamically stabilizes the lattices by both keeping the origami in a thin layer so that their local concentration is increased and orienting the origami so that their corners are better aligned for bonding than origami undergoing 3D diffusion in solution. Put another way, surface confinement encourages lattice formation by partially paying the translational and rotational entropic costs of fixing an origami monomer into a lattice. Figure 2: DNA origami checkerboard lattices self-assembled by surface diffusion. ( a , b ) Before assembly ( a ) no lattices are observed by AFM, but after the surface diffusion protocol ( b ) 98.6% of rectangles ( n =2,380) have been incorporated into lattices. Images in a and b are not from the same position on the mica surface, but are representative before/after images. ( c , d ) Consecutive AFM images show attachment events of origami to lattices (orange circles), detachment events (green triangles), movements of individual origami or small lattices which appear or disappear between frames (blue rectangles) and structures dragged by the AFM tip (yellow arrows). All images are 10 μm × 10 μm. Full size image Figure 2c,d shows consecutive AFM images taken during the surface diffusion step. This image pair captured a few attachment events of rectangles to lattices (orange circles) and a few detachment events (green triangles). The images also reveal movement (blue squares) of monomers and dimers, which either disappear after the first scan or appear in the second scan at spots where no origami were previously observed. The fact that many origami in Fig. 2c,d appear to be partially imaged or have an irregular shape reflects the increased mobility of individual origami. Linear traces (yellow arrows) may indicate the path of individual rectangles getting dragged by the AFM tip; in Fig. 2d , for which AFM conditions may have changed slightly, traces can be up to several microns long. Such artifacts suggest that lattice formation proceeds via the motion of origami that, while loosely bound to the surface, do not completely leave it (more evidence below). Control experiments To understand which aspects of our protocol were necessary and sufficient for lattice formation, and to test the hypothesis that the assembly is restricted to 2D, we carried out a series of systematic control experiments changing exactly one factor at a time ( Figs 3 and 4a ). Above we noted that no lattices were observed by AFM for origami samples deposited directly from their formation buffer, but it remained possible that addition of 700 mM Na + and 40 °C incubation during Step 2 would have been sufficient for lattice formation to occur in solution, without the mica surface. We thus replicated Step 2 in a test tube, and observed that no lattices were formed ( Fig. 3a ), confirming mica’s role in lattice formation. Next, we asked whether Na + was necessary for lattice formation, by repeating Step 2 without the addition of Na + , and observed ( Fig. 3b ) that no lattices formed. We further observed that origami can be successfully synthesized without Mg 2+ (recently reported elsewhere [38] ), which allowed us to ask an analogous question about the necessity of Mg 2+ for lattice formation. Surprisingly, after forming and depositing origami in pure Na + (0.75 M, under which buffer imaging of origami is impossible) we found, post-incubation and immobilization, that small lattices were formed (2.7±1.1 origami per lattice, 489 origami) but only 65% of the origami were incorporated into lattices ( Fig. 4a ). This suggests that origami bind weakly to mica, even in the complete absence of added divalent cations (or perhaps the mica we used contains traces of Mg 2+ , Zn 2+ or other divalents), and that Mg 2+ was important for creating larger lattices like those in Fig. 2b . Heating during the incubation step was found to be optional for lattice formation ( Fig. 3c ), as we observed small to medium-sized lattices (3.4±1.8 origami per lattice, 275 origami) and a high extent of lattice incorporation (92%); we suggest that heating may encourage formation of larger lattices, but have not explored this extensively. 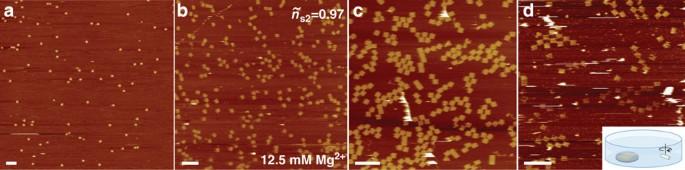Figure 3: Control experiments. (a) Mica-free condition, in which origami were subjected to Step 2 incubation in a test tube. (b) Na+-free condition, performed in TAE/Mg2+. (c) Heat-free condition. (d) Large-volume condition, wherein the entire mica substrate was immersed in a 6 ml reservoir of Na+solution during Step 2 (inset shows a schematic of the experimental setup). Scale bars, 500 nm. Figure 3: Control experiments. ( a ) Mica-free condition, in which origami were subjected to Step 2 incubation in a test tube. ( b ) Na + -free condition, performed in TAE/Mg 2+ . ( c ) Heat-free condition. ( d ) Large-volume condition, wherein the entire mica substrate was immersed in a 6 ml reservoir of Na + solution during Step 2 (inset shows a schematic of the experimental setup). Scale bars, 500 nm. 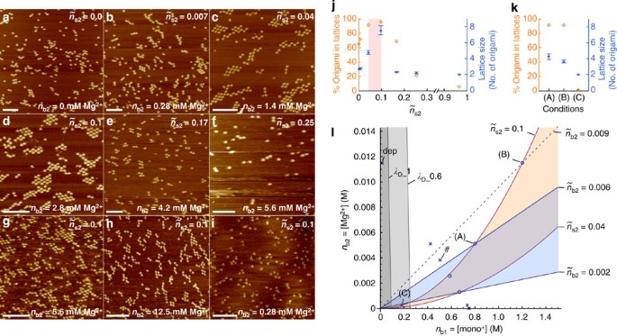Figure 4:Lattice formation as a function of varying Mg2+and Na+concentrations during the surface diffusion step. (a–f) AFM data after deposition and assembly using buffers giving the following fractional surface densities of Mg2+: (a) 0 (Mg2+-free, Na+-only, condition), (b) 0.007, (c) 0.04, (d) 0.1, (e) 0.17, and (f) 0.25. (g–i) AFM data for additional test conditions (A) through (C), respectively, all of which had. (j) The extent of lattice incorporation (orange diamonds, percentage of origami found in lattices) and lattice size (blue-filled diamonds) with respect to thevalues examined in (a–f) and assembly under the deposition condition. Error bars indicate standard error (n=489, 528, 1,133, 1,196, 382, 167 and 209, in order). The pink area indicates the optimal working regime, with lattice incorporation of >90%. (k) Lattice incorporation and lattice size for additional test conditions, (A) through (C), corresponding to (g–i), respectively (n=495, 396 and 210). (l) Plot of conditions with respect to bulk ion concentrations,nb2andnb1, highlighting thatbetter correlates with high lattice incorporation rates than does its bulk counterpart, except in the limit of high Debye length,λD. Red parabolas denote constantvalues, blue lines denote constantvalues, and grey lines denote constantλDvalues. Shaded areas highlight continuous ranges of values between contours of constant(orange),(blue) andλD(grey). Circles denote conditions with high lattice incorporation rates (>90%); the remaining conditions (‘ × ’) had significantly lower lattice incorporation rates. A single condition (‘#’) with a significantly lower lattice incorporation rate (<70%) prevents the blue shaded area from being extended to the blue dotted line, and demonstrates that no single continuous range ofvalues can capture the working regime. (A), (B) and (C) mark conditions for the additionalexperiments. ‘dep’ indicates the deposition condition. Scale bars, 1 μm. Full size image Figure 4: Lattice formation as a function of varying Mg 2+ and Na + concentrations during the surface diffusion step. ( a – f ) AFM data after deposition and assembly using buffers giving the following fractional surface densities of Mg 2+ : ( a ) 0 (Mg 2+ -free, Na + -only, condition), ( b ) 0.007, ( c ) 0.04, ( d ) 0.1, ( e ) 0.17, and ( f ) 0.25. ( g – i ) AFM data for additional test conditions (A) through (C), respectively, all of which had . ( j ) The extent of lattice incorporation (orange diamonds, percentage of origami found in lattices) and lattice size (blue-filled diamonds) with respect to the values examined in ( a – f ) and assembly under the deposition condition . Error bars indicate standard error ( n =489, 528, 1,133, 1,196, 382, 167 and 209, in order). The pink area indicates the optimal working regime, with lattice incorporation of >90%. ( k ) Lattice incorporation and lattice size for additional test conditions, (A) through (C), corresponding to ( g – i ), respectively ( n =495, 396 and 210). ( l ) Plot of conditions with respect to bulk ion concentrations, n b2 and n b1 , highlighting that better correlates with high lattice incorporation rates than does its bulk counterpart , except in the limit of high Debye length, λ D . Red parabolas denote constant values, blue lines denote constant values, and grey lines denote constant λ D values. Shaded areas highlight continuous ranges of values between contours of constant (orange), (blue) and λ D (grey). Circles denote conditions with high lattice incorporation rates (>90%); the remaining conditions (‘ × ’) had significantly lower lattice incorporation rates. A single condition (‘#’) with a significantly lower lattice incorporation rate (<70%) prevents the blue shaded area from being extended to the blue dotted line, and demonstrates that no single continuous range of values can capture the working regime. (A), (B) and (C) mark conditions for the additional experiments. ‘dep’ indicates the deposition condition. Scale bars, 1 μm. Full size image We next asked whether the origami are truly confined in 2D on the surface during assembly. Our observation that 4 h incubation in a test tube does not result in lattices confirms the requirement of mica for lattice formation, but it might still be possible that origami move primarily by jumping into the solution, diffusing in 3D and later returning to the surface. To test this hypothesis, we performed the deposition step as usual, but then immersed the entire mica substrate in large bath of NaCl solution in a Petri dish (6 ml, ~150 times the usual volume used for Step 2, and ~1,200 times the volume of the origami solution deposited; see Fig. 3d inset). We also agitated the solution with a magnetic stir bar throughout the incubation to ensure that the solution was well-circulated. Under such conditions, our expectation was that if origami rectangles did leave the surface during assembly, most origami would have been lost into solution and significantly fewer would have been observed after immobilization. Instead, numerous small to medium-sized lattices were observed (along with greater-than-usual surface contamination, Fig. 3d ), suggesting that origami are confined to the surface during lattice formation. Potential mechanisms for binding and surface diffusion The lattice-formation phenomenon we describe depends on two different DNA–mica binding regimes: strong DNA–mica binding for the deposition and immobilization steps, and weak DNA–mica binding for the surface diffusion step. Below we review what is known about cation-dependent strong DNA–mica binding, and strong-to-weak DNA–mica binding transitions and explore how it might apply to lattice formation. Mica is a layered mineral with a negative surface charge, and DNA is a negatively charged polymer. Thus divalent cations, such as Mg 2+ and Ni 2+ , are often described as mediating the binding of DNA to mica by bridging the negative charges on the DNA backbone and those on the mica [29] , [31] , [35] , [36] , [39] . This is a great simplification of divalent-cation-mediated DNA–mica binding, since the strength of binding for a particular cation concentration depends strongly on the identity of the cation, the size and geometry of the DNA object in question and the method of sample preparation. We know of no reported equilibrium constants for DNA–mica binding as a function of cation type and DNA structure, but one can get an idea of the binding strength by considering what is visible by AFM imaging under buffer, during which the AFM tip can sweep loosely bound DNA objects aside rendering them invisible. For example, a daily experience in our lab is that 12.5 mM Mg 2+ is insufficient to provide stable buffer imaging of 14.5 kilonucleotide (knt) linear dsDNA that often occurs as a minor impurity of m13 dsDNA in origami preparations. Similar experience with dsDNA in many labs has led to the idea that Mg 2+ binds DNA to mica but only very weakly [29] , [32] . However, 12.5 mM Mg 2+ provides for stable buffer imaging of 14.5 knt single-layer DNA origami such as rectangles or triangles, but not for structures which present areas significantly smaller than the 7,000 nm 2 area of a 14.5 knt single-layer origami, such as a ~5 knt single-layer rectangle [1] . In general, for a given buffer condition, 2D DNA nanostructures bind mica more strongly than linear dsDNA with the same number of nucleotides, and larger and/or flatter objects bind more strongly than smaller and/or 3D ones. On the other hand, some divalent cations mediate strong binding of even small dsDNAs at millimolar concentrations: just 2 mM of the cations Ni 2+ , Co 2+ or Zn 2+ allow stable AFM imaging of 0.6 knt dsDNA under buffer, whereas Mg 2+ , Hg 2+ and Cd 2+ do not [29] . Ni 2+ apparently binds to mica so strongly that Ni 2+ pretreatment of the surface is all that is necessary to immobilize short dsDNA [31] , [40] . The idiosyncratic properties of each divalent metal cation with respect to DNA binding to mica have been partially attributed to cationic radius or enthalpies of hydration [29] or specific complexation of the ions with DNA or mica [31] , but no theory consistently explaining the behaviour of all divalent cations seems to exist. Further complicating matters, monovalent cations commonly present in buffer solutions such as Na + , K + or TrisH + can decrease the interaction of divalent cations with DNA and mica. [31] , [32] , [35] , [36] For particular cations, for linear dsDNA, three studies by the same group have been successful in explaining strong-to-weak binding transitions of particular relevance to our system [31] , [32] , [40] . In the first study [31] , the effect of competition between Mg 2+ and Na + cations on the end-to-end distances of 1.4 knt linear dsDNA was described using a combination of the charge screening length (Debye length, λ D ) and the fractional surface density of divalent cations, . End-to-end distance was taken as a surrogate for binding strength, with greater distance implying weaker binding. For conditions of low ionic strength ( I <0.1 M), under which λ D is larger than the average distance between two charges on DNA or mica (~1 nm), it was noted that divalent cations sandwiched between DNA and mica will be significantly affected by each other and by the negative charges on the DNA and mica. In this regime, it was proposed that correlations between divalent cations result in a staggered up/down configuration, with alternating Mg 2+ ions associated with the surface and with the DNA. This ‘ion correlation model’ predicts short-range attraction of DNA to the mica surface and it defines an ionic-strength-independent mode of DNA–mica binding. As predicted, for a given , end-to-end distance was roughly constant for I <0.1 M. Further, was well-correlated with end-to-end distance, with lower corresponding to greater distance. For higher ionic strength ( I ≈0.1 M), the Debye length drops below the Bjerrum length, the distance for which the electrostatic potential of two charges equals their thermal energy (0.7 nm in water), and thus it was assumed that thermal energy would disrupt the staggered ion correlations. This would predict a qualitative change in the mode of DNA binding to the surface and a weakening of the binding strength. Indeed, an abrupt increase in end-to-end distance was observed at I ≈0.1 M for two different values of . In summary, both Debye length and influenced binding strength, but for a given , Debye length governed a strong-to-weak binding transition at I ≈0.1 M. In a second study [40] , the surface diffusion rate of the same 1.4 knt dsDNA was related to electrostatic surface friction, which was in turn related to the strength of ion correlations. Ni 2+ -treatment of mica prevented geometric rearrangement of highly entangled DNA, which otherwise was able to untangle. Thus surface diffusion-mediated DNA rearrangement (in this sense an analogue of lattice formation) was found to be governed by a strong-to-weak binding transition based on ion correlations. In a third study [32] , a transition in DNA–mica binding mode from ‘adsorption’ (in which circular 2.6 knt DNAs were tightly bound and spread out on the surface) to ‘nonadsorption’ (in which DNAs remained loosely bound to the surface) was found to occur consistently as decreased through ~0.65 (estimated from Fig. 3 of ref. 32 ) over a wide range of Mg 2+ and Na + conditions at ionic strengths up to ~1 M. This suggests that can, by itself, capture strong-to-weak binding transitions in DNA–mica interactions. Our particular approach to inducing 2D assembly is motivated by such studies and thus it is natural to examine whether the Debye-length-dependent ion correlation model or a simple single -demarked strong-to-weak binding transition can capture conditions for origami lattice formation. During origami deposition (Step 1), λ D ~1.2 nm and so the ion correlation model, with its strongly localized divalent cations, is consistent with the observed immobility of DNA origami and inability to form lattices under this condition. With the addition of Na + during surface diffusion (Step 2), the solution has an ionic strength of ~0.7 M and the Debye length is estimated to be ~0.34 nm. Thus, in theory, thermal energy should perturb the ~1 nm-scale correlations between the Mg 2+ bridging the DNA and mica, weakening the overall binding strength, which is consistent with our observation that the origami have increased mobility and rearrange to form lattices. However, because DNA origami bind mica so much more strongly than linear DNA, we find (below) that the lattice-forming regime starts at much higher ionic strength and lower Debye length ( I >0.4 M and λ D ≲ 0.45 nm) than would be naively predicted by the ion correlation model developed for linear DNA. The idea that , the fractional surface density of Mg 2+ , could alone predict the strong-to-weak transition which enables surface diffusion in our system is attractive for two reasons. First, as explained below, is a very natural quantity for predicting DNA–mica binding behaviour. Second, it would provide a unifying picture for strong-to-weak DNA–mica binding phase transitions. For any geometry, whether linear dsDNA or 2D DNA origami, there might exist an (potentially different, depending on geometry) at which DNA structures go from an immobile state to a weakly bound state compatible with surface diffusion. The fact that 2D DNA origami bind mica more strongly than dsDNA would predict that the critical for origami would be less than that observed for the particular circular dsDNA reported (0.65). The lattice incorporation rate, which begins to rise as falls below ~0.2, is consistent with this prediction. However, lattice incorporation is not a direct measure of surface diffusion, and optimal lattice incorporation appears to require more than merely high rates of surface diffusion, because lattice incorporation begins to drop off as falls below 0.04. Thus below we find that lattice formation follows a somewhat complex rule: small Debye length permits the formation of lattice, within a range of optimal values. Effect of ionic conditions on lattice formation Having explored a variety of extremal conditions in our control experiments, we sought to optimize conditions for lattice assembly and gain an understanding of which experimental parameters best explained the optimal working regime. Clearly Mg 2+ and Na + concentrations both play a role, but depending on the mechanism of binding and surface diffusion, the extent of lattice incorporation might correlate best with just the Mg 2+ concentration, just the Na + concentration or a parameter which is a function of both Mg 2+ and Na + concentrations such as ionic strength or Debye length. Of particular interest are parameters involving the concentration of different cations at the surface, which can be very different than those in the bulk. Let n s be the total surface concentration of neutralizing cations, and n s z be the surface concentration of cations having valence z . Then we define the fractional surface densities of the monovalent and divalent cations, and as in ref. 41 : In addition to the above-mentioned studies [31] , [32] which support the importance of , the parameter has intrinsic properties which suggest it should correlate well with DNA–mica interactions. For strongly ionizing negative surfaces such as mica and DNA, the total surface concentration of cations ( n s ) is assumed to be constant regardless of cation valence or bulk concentration of cations. This somewhat counterintuitive result arises because the volume used for calculating n s is defined by λ z , the characteristic distance at which the electric potential energy of a cation equals the thermal energy [41] , which depends on the cation valence. The constancy of n s (estimated to be 16 M for mica [31] ) implies that a particular value of corresponds in a one-to-one manner with a particular pair of Mg 2+ and Na + surface concentrations, rather than all possible pairs of Mg 2+ and Na + surface concentrations having a ratio equal to that value, as might be naively expected. Other parameters do not have a one-to-one relationship with surface concentrations: for example, a single value of the bulk solution fraction of divalents, , can map to multiple pairs of Mg 2+ and Na + surface concentrations. Thus the parameter most simply captures the state of mixed layers of Mg 2+ and Na + near a mica surface and we chose to explore the effect of on lattice formation. The competition between divalent and monovalent cations for occupancy in the thin layer above a negatively charged surface is modelled by the Poisson–Boltzmann equation, which allows the calculation [31] , [42] of effective surface concentrations for the monovalent cations ( n s1 ) and the divalent cations ( n s2 ) given the bulk concentrations n b1 and n b2 and the electrostatic potential at the surface ( ψ ): where e is the elementary charge, k B is the Boltzmann constant, and T is the temperature. Since and satisfy the relation we can obtain the fractional surface densities, and , from corresponding bulk concentrations, without knowing the surface potential by combining (1)–(4) to yield a simple quadratic equation [31] , [42] . Here we give calculated for mica, whereas ref. 31 gives calculated for DNA. See Supplementary Note 3 for a comparison. Here we give the formal [Mg 2+ ] rather than an effective [Mg 2+ ], which takes EDTA chelation of Mg 2+ into account, and refer to [Na + ] when [mono + ] would be more precise. Supplementary Note 3 uses the more precise quantities. has a one-to-one correspondence with n b2 / n b1 2 =[Mg 2+ ]/[Na + ] 2 and so everything presented here can be cast in terms of this bulk solution parameter if desired. By mixing different ratios of origami formed in either 0.75 M Na + or TAE/Mg 2+ and subjecting them to surface diffusion, we observed assembly under a variety of conditions ranging from to ( Fig. 4a–f up to , shown in Fig. 3b , results are summarized in Fig. 4j , see Supplementary Note 4 for more discussion). This series of conditions was chosen so that both the absolute concentrations of Mg 2+ and Na + , as well as , would correspond to conditions at important steps in our standard protocol. In particular, the condition corresponds to Step 2 under the standard assembly protocol, and the condition corresponds to the initial deposition Step 1. We observed that lattice size and percent of monomers incorporated into lattices rose quickly until and then fell sharply by . Our conclusion was that first, a certain surface fraction of Mg 2+ is important for lattice formation, perhaps by increasing confinement to the surface, and second, given too much Mg 2+ , above a certain surface fraction , origami are too immobile to rearrange to form large lattices. We declared conditions for which the extent of lattice incorporation was >90% to be the working regime for our assembly protocol, which corresponds to a single continuous range of values . We note that average lattice size was sometimes inconsistent over a single sample (shown later), and across different experimental conditions it exhibited a smaller fold-difference (4 ×) than lattice incorporation (>50 ×). These observations motivated our use of lattice incorporation to compare and other parameters. For the series of conditions in Fig. 4j , we examined whether other parameters might be equally-well used to define the working regime with a single continuous range of values. The top plots of Supplementary Fig. 1b–f show that for all other parameters which we examined ( n b2 =effective [Mg 2+ ], n b1 =[monovalents + ], the bulk solution fraction of divalents , ionic strength I and Debye length λ D ) it was possible to define a continuous working regime (for example, 0.60 M≤ I ≤0.67 M). To further distinguish which parameter best captures the working regime for lattice formation, we carried out experiments for additional extreme conditions at which was constant, but other parameters varied. In particular, we chose three conditions for which , the value which gave the greatest lattice incorporation in previous tests for a condition which had an intermediate amount of Mg 2+ ( Fig. 4d ). Two higher-Mg 2+ conditions, (A) and (B), were chosen so that their bulk Mg 2+ concentration corresponded to that in earlier tests for which there was poor ( Fig. 4f ) or almost no lattice incorporation ( Fig. 3b , equivalent to the deposition condition). Condition (C) was chosen to correspond to a previous lower-Mg 2+ condition ( Fig. 4b ), which exhibited moderate (~70%) lattice incorporation. Na + concentrations were adjusted up (conditions (A) and (B)) or down (condition (C)) to achieve . Figure 4g–i shows AFM data and Fig. 4k summarizes results. Conditions (A) and (B) gave >90% lattice incorporation rates ( Fig. 4k ). For all parameters besides , these data preclude the definition of a working regime with a single continuous range of values. After , the best correlating parameter is , which is disqualified by a single moderate (~70%) lattice-forming condition between values yielding excellent (≥90%) lattice formation ( Supplementary Fig. 1d , bottom). Figure 4l provides a comparison of how well and correlate with the data, and provides a map for which conditions should be tested in the future to further differentiate them. Ionic strength, Debye length and bulk monovalent concentration are more strongly disqualified by the presence of two moderate lattice-forming conditions between parameter values yielding excellent lattice formation ( Supplementary Fig. 1c,e,f , bottom). Bulk Mg 2+ concentration is the worst correlating parameter, exhibiting two [Mg 2+ ] values for which both poor (≤20%) and excellent lattice formation were observed ( Supplementary Fig. 1b , bottom). Condition (B) starkly shows that even a very high bulk Mg 2+ , of 12.5 mM, which renders origami completely immobile in the low-monovalent (15 mM) deposition buffer ( Fig. 3b ), can allow surface diffusion and lattice formation ( Fig. 4h ) when combined with a suitably high (1.2 M) concentration of monovalent Na + cations. Seen through the lens of this is unsurprising. Even though the condition in Fig. 4d , and conditions (A) and (B) span a large range of bulk Mg 2+ from 2.8 to 12.5 mM, they all have exactly the same surface fraction of Mg 2+ (0.1), and hence the same absolute Mg 2+ concentration (1.6 M) on the surface (see Supplementary Fig. 2 ). The extremely poor (<1%) lattice formation observed at condition (C), a low Mg 2+ (0.28 mM) and low Na + (0.18 M) condition, shows that does not completely capture the assembly process. Monovalent concentration, ionic strength and Debye length group condition (C) with other poor lattice-forming conditions, far away from other better lattice-forming conditions, and thus better explain this datum ( Supplementary Fig. 1c,e,f bottom) than do and , which place condition (C) between good and excellent lattice-forming conditions. Condition (C) is differentiated from all other lattice-forming conditions in that its Debye length (0.70 nm) is both much higher than any conditions for which any lattice formation was observed ( λ D of 0.24 to 0.43; see Supplementary Table 1 for all values, and Supplementary Note 2 for calculations), and much closer to the charge separation distance of Mg 2+ ions in the ion correlation model (~1 nm). An alternative explanation for poor lattice formation under condition (C) is that the low ionic strength weakens the stacking bonds themselves. To exclude the possibility that buffer-dependent changes to the strength of stacking bonds was changing the rates of lattice incorporation, we performed solution experiments, which verified that the strength of stacking bonds were minimially effected for ionic conditions which gave low lattice incorporation rates ( Supplementary Note 5 ). Putting our observations together, high lattice incorporation rates require that two criteria be met: first, ionic strength must be high enough ( I >0.4 M) that the Debye length is much shorter ( λ D ≲ 0.45 nm) than the Mg 2+ charge separation distance, and second, must be in the range 0.04 to 0.1. While the first criterion suggests a role for ion correlations, it is not quantitatively compatible with the ion correlation model previously reported for linear dsDNA [31] . We emphasize that this is unsurprising given the much stronger binding of DNA origami—perhaps a 2D ion correlation model, with ions exhibiting staggered configurations in 2D, would explain both the low Mg 2+ requirement for origami-mica binding and the high-ionic strength requirement for origami surface diffusion/lattice formation. The onset of lattice formation at , is lower than the previously observed strong-to-weak DNA–mica binding transition [32] , but again this is understandable in terms of stronger origami binding. Given the picture of a single strong-to-weak transition, there is no reason to expect that surface diffusion should ever decrease, once it has fallen below the putative transition at , and thus one might expect high lattice incorporation down to . But while lattices form in an absence of Mg 2+ , at , they exhibit only moderate lattice incorporation (~65%). This suggests that while binding strength cannot be too strong, it must at least exceed some threshhold, so at least some Mg 2+ is required for high lattice incorporation rates—as noted in the original motivation for our protocol, this may serve to pay entropic costs associated with concentrating and orienting the origami at the surface. Another possibility relates to the origami’s 3D geometry: origami are highly twisted in solution. As binding strength increases, origami may become increasingly flat and steric hindrance to bond formation may decrease. It may be that the rising-and-falling behaviour of lattice incorporation (as rises) can be explained as the result of an initial increase in lattice incorporation, as initial flattening overcomes steric hindrance, which is followed by a decrease in lattice incorporation, as further flattening increases the bound area of the origami, electrostatic friction increases and surface diffusion decreases. We do not have direct evidence of this, but later we report experiments which suggest that origami twist is critical to the surface-dependence of lattice formation. Effects of origami design The predominant product of surface diffusion is 2D lattices—yet the geometric arrangement of blunt ends at the rectangle’s corners are also compatible with 1D linear chains ( Supplementary Note 6 ). We initially hypothesized that the bias towards lattices might be due to non-uniformity of the blunt-end sequences that occur at the corners of the origami ( Supplementary Fig. 3 ), which could result in preferential bond orientations. However, control experiments with uniform sequences still predominantly yielded lattices ( Supplementary Fig. 4 ). Instead we found that global twist of the origami and distortion induced by the twist governed the assembly behaviour: while twisted origami favored the formation of 2D lattices, twist-reduced origami allowed the formation of linear chains ( Supplementary Fig. 5 ). To search for optimal lattice formation as a function of origami design, we varied bond strength and size ( Supplementary Note 7 ) and found that larger, stronger bonds ( N =5 and N =7) performed worse ( Supplementary Fig. 6 ). In solution, they allowed the formation of linear chains, demonstrating that stronger stacking bonds can better overcome the distortion of highly twisted rectangles. Upon surface diffusion, diagonal chains predominated over 2D lattices. We believe that this is because larger stacking bonds provide greater steric constraints which are incompatible with the formation of checkerboard lattices, while still allowing diagonal bonds to form ( Supplementary Fig. 7 ). Effect of mica inhomogeneities Our original desire was to optimize assembly conditions to achieve very large lattices. While we could routinely generate samples for which >95% of origami were incorporated into lattices, and some samples exhibited lattices comprising >50 origami, we found that we could not find cation concentrations, annealing profiles or origami concentrations, which would reproducibly yield such large lattices. While the origami regularly formed lattices with a roughly 1:1 length:width aspect ratio, on rare occasions they would yield lattices with aspect ratios in excess of 20:1. These results puzzled us until we imaged the sample presented in Fig. 5 and Supplementary Fig. 8 , in which lattices of numerous aspect ratios and sizes appear, from single-origami-width diagonal chains extending for dozens of origami, to roughly 8 × 8 lattices. 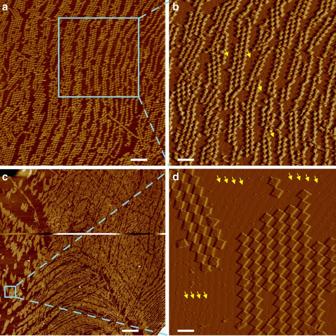Figure 5: Formation of checkerboard lattices of varying aspect ratio on a single mica surface. (a,b) Origami checkerboard lattices whose edges appear to follow ‘domain boundaries’ of a mica surface. The zoom-in tapping amplitude image (b) of the boxed area inareveals some of the putative domain boundaries (indicated by arrows). (c) A large-area AFM image (30 μm × 30 μm) that shows large regions of distinct lattice morphology. (d) A zoom-in tapping amplitude image of the boxed area inc, from a region with particularly large, well-separated, single-domain lattices. The zoom shows narrow (roughly origami-sized), long domains. Boundaries between domains appear as parallel lines and are again indicated by arrows. These rectangles had ‘GC’ blunt ends. Scale bars, (a) 1 μm, (b) 500 nm, (c) 3 μm and (d) 200 nm. Figure 5: Formation of checkerboard lattices of varying aspect ratio on a single mica surface. ( a , b ) Origami checkerboard lattices whose edges appear to follow ‘domain boundaries’ of a mica surface. The zoom-in tapping amplitude image ( b ) of the boxed area in a reveals some of the putative domain boundaries (indicated by arrows). ( c ) A large-area AFM image (30 μm × 30 μm) that shows large regions of distinct lattice morphology. ( d ) A zoom-in tapping amplitude image of the boxed area in c , from a region with particularly large, well-separated, single-domain lattices. The zoom shows narrow (roughly origami-sized), long domains. Boundaries between domains appear as parallel lines and are again indicated by arrows. These rectangles had ‘GC’ blunt ends. Scale bars, ( a ) 1 μm, ( b ) 500 nm, ( c ) 3 μm and ( d ) 200 nm. Full size image Surprisingly, different lattice forms appeared to dominate in different areas of the mica, as if the mica surface was nonuniform. Upon zooming in we observed patterns of fine parallel lines (yellow arrows, Fig. 5b,d ) that did not correlate to the hexagonal lattice of the mica structure. The lines define ‘domain boundaries’ whose width appears to dictate the observed pattern of origami lattice formation. Where domains are wide, origami lattices are large and densely packed. As the width of the domains decreases, the width of origami lattices decreases, down to the width of a single origami chain ( Fig. 5a,b ). Where the domain width is roughly the same as, or slightly smaller than, the period of origami, lattices are large again, and the largest lattices observed were obtained in such regions. We hypothesize that the observed domains correlate with charge distribution, and that the origami are absent at domain boundaries because they are less sticky, potentially presenting less negative charge for the binding of Mg 2+ cations. Areas with domains whose width is roughly the period of origami in lattices ( Fig. 5d ) may have allowed larger single origami lattices because these lattices may nucleate infrequently (since the mica is on average less sticky than in the middle of a wider domain), or the periodic pattern of the domains may align monomers and lattices in a coherent manner (note the alignment of lattices with the domain boundaries in Fig. 5d ). Although we have not conclusively excluded alternative mechanisms such as solution flow for the observed pattern of origami lattices, the presence of observable, correlated features in the mica surface, strongly implicates the mica surface as a determinant of lattice size and morphology. We note that while lattice size and morphology is highly nonuniform in the sample presented in Fig. 5 , the extent of lattice incorporation is constant and high (~99%) for both regions of densely packed elongate lattices (for example, the right half of Fig. 5b ) and sparse but more compact lattices (for example, Fig. 5d ) which is further support for our use of the extent of lattice incorporation rather than lattice size in mapping the optimal conditions for lattice formation. We have been unable to find literature that reports similar domains in mica surfaces, and we do not have a satisfactory model for their atomic structure. However, we note that muscovite mica is a complex mineral with highly varied chemical composition [43] and it has a high degree of disorder at certain lattice sites. For example, ‘tetrahedral sites’ [44] , [45] can randomly host Si 4+ or Al 3+ and ‘octahedral sites’ [46] which are mostly occupied by Al 3+ can also host Mg 2+ or Fe 2+ . It is the substitution of Si 4+ by Al 3+ at tetrahedral sites that gives layers of muscovite mica their net negative charge. Such sites are generally thought of as disordered (as measured by crystallography) and thus random substitution of these ions would result in uniform charge. However, Bailey [45] reviews evidence suggesting short-range order at tetrahedral sites, including the idea that chains of Si and Al may alternate, or that there might be other wave-like distortions of the mica lattice. While domains such as those in Fig. 5 were not always observed, we believe that such inhomogeneities of mica surfaces may limit our control over the size and morphology of origami lattices. With respect to our technological goal, our method has succeeded in reproducible growth of DNA lattices, averaging up to eight origami in size, over large areas of a mica surface. It is fast, simple and unlike previous surface-based self-assembly of small DNA tiles [26] , [27] , [28] our method can operate isothermally, which may be advantageous if the method is used to organize temperature-sensitive components such as proteins. Formation of larger lattices involving 50 or more tiles is, so far, dependent on irreproducible properties of inhomogeneous mica surfaces. However, a combination of directed self-assembly and surface diffusion might allow the creation of large, aligned lattices on the wafer scale. Because we observe that the largest single-domain lattices form and align to patterns of parallel domains whose period roughly matches the size of individual origami ( Fig. 5d ), it is possible that analogous chemical patterning of a silicon dioxide substrate, with parallel stripes of alternating chemical character, would achieve reproducible fabrication of large lattices. There is precedent for similar types of patterning. Weak interactions between block copolymers and chemically patterned substrates have been successfully used to create large-scale low-defect periodic patterns [47] . Here the surface-dependent formation of lattices depended on the particular use of rectangular origami of high twist, which prevented formation of stacking bonds in solution and dictated the formation of checkerboard lattices of ~90 nm period with rectangular vacancies. Rather than relying on twist to keep origami as monomers in solution, the strength of the stacking interactions is easily weakened to achieve the same effect with flattened origami of arbitrary shape. In general, other shapes, such as squares or crosses having bonds on all four sides, could easily be used to achieve lattice geometries other than checkerboards, of different lattice periods, with or without vacancies. Further, the origami support internal patterning [1] , which would allow periodic patterns down to ~6 nm. We do believe that the strong-to-weak DNA–mica binding transition will be affected by origami geometry, and thus we expect that flatter origami might require lower and smaller origami might allow the use of higher for optimal lattice formation. When dealing with weak binding of a DNA nanostructure to mica, common experimental practice has been to simply add more Mg 2+ or Ni 2+ , without regard to the role of monovalent cations. This work shows that the bulk Mg 2+ concentration cannot be used as the sole predictor of the behaviour of DNA origami on mica. In fact, the phenomena observed in this work cannot be observed by simply varying Mg 2+ concentration, as previous works studying the surface-mediated assembly of small DNA tiles have done [28] . Further this work demonstrates that one cannot simply translate models and results achieved for linear dsDNA to artificial DNA nanostructures since DNA size and geometry have profound effects on DNA–mica binding. For now, key biophysical experiments, like those presented here, will have to be repeated to calibrate the behaviour of each DNA nanostructure under study. Ultimately, a comprehensive theory of DNA nanostructure–mica binding—one which takes into account cation type, nanostructure geometry and details of surface treatment—will have to be constructed. Origami preparation Origami designs were adopted from previous studies [1] , [33] . Strand and sequence diagrams can be found in Supplementary Fig. 9 , and sequence lists are supplied as Supplementary Data . Single-stranded M13mp18 DNA (scaffold strand) was purchased from New England Biolabs (Catalogue #N4040S) or Bayou Biolabs (Catalogue #P-107) and staple strands were obtained unpurified from Integrated DNA Technologies in water at 150 μM. Scaffold and staples were mixed together at target concentrations of ~2 nM and ~75 nM, respectively, in TAE (40 mM Tris acetate, 1 mM EDTA) buffer with 12.5 mM magnesium acetate (TAE/Mg 2+ ). Origami mixtures were kept at 90 °C for 5 min and annealed from 90 to 20 °C at −1 °C min −1 . For origami synthesized in Na + solution, 0.75 M NaCl was substituted for 1 × TAE buffer. Surface diffusion assembly protocol Step 1: rectangles were deposited from a 2 nM origami solution onto a freshly cleaved mica substrate (Ted Pella). Typically a 20 μl drop of buffer solution was added to the mica first, to which 5 μl of origami solution was added, before letting the sample sit for 20 min inside a small (35 mm) Petri dish with a lid (to prevent evaporation and contamination). Step 2: the buffer was exchanged by slowly removing ~20 μl of the TAE/Mg 2+ buffer via pipette (origami were strongly bound to the surface and not perturbed by fluid flow; the mica substrate was slightly tilted—this facilitated removal of liquid from the lower edge of mica), leaving ~5 μl of the buffer on the mica surface. Next, 40 μl of 0.75 M NaCl solution was added. Finally, the Petri dish was sealed with parafilm, placed inside a temperature-controlled box (Coy Laboratory Products Inc.) and incubated at 40 °C for ~4 h. Step 3: after incubation, 5 μl of 10 mM nickel acetate solution was added on top of the substrate (while keeping the substrate within the 40 °C box) to ‘freeze’ product structures. After 5 min, the NaCl buffer was exchanged back to TAE/Mg 2+ and the substrate was removed from the box for AFM analysis. Atomic force microscopy Samples for AFM imaging before the surface diffusion protocol were prepared by depositing 5 μl of the origami solution with 20 μl of TAE/Mg 2+ buffer onto freshly cleaved mica (Ted Pella). Clean buffer solution was deposited first and the origami solution was added on top (for concentrated samples we felt that this procedure minimized spatial variation in the density of origami on the mica.) AFM images were taken under buffer in fluid tapping mode with a Multimode AFM (Veeco Metrology Group, now Bruker AXS) using a Nanoscope IIIa controller. Silicon nitride cantilevers with 2 nm radius silicon tips were used (the ‘short, fat’ A cantilever on SNL probes from Bruker). For sequential scans taken during surface diffusion (for example, Fig. 2c,d ), tip-sample interaction was reduced by lowering the tapping drive amplitude and optimizing the amplitude set-point. How to cite this article : Woo, S. and Rothemund, P. W. K. Self-assembly of two-dimensional DNA origami lattices using cation-controlled surface diffusion. Nat. Commun. 5:4889 doi: 10.1038/ncomms5889 (2014).